The vectorial control of magnetization by light Application of coherent light–matter interactions has recently been extended to the ultrafast control of magnetization. An important but unrealized technique is the manipulation of magnetization vector motion to make it follow an arbitrarily designed multidimensional trajectory. Here we demonstrate a full manipulation of two-dimensional magnetic oscillations in antiferromagnetic NiO with a pair of polarization-twisted femtosecond laser pulses. We employ Raman-type nonlinear optical processes, wherein magnetic oscillations are impulsively induced with a controlled initial phase. Their azimuthal angle follows well-defined selection rules that have been determined by the symmetries of the materials. We emphasize that the temporal variation of the laser-pulse polarization angle enables us to control the phase and amplitude of the two degenerate modes, independently. These results lead to a new concept of the vectorial control of magnetization by light. Recent advances in ultrashort-pulsed laser technology have enabled the ultrafast control of magnetization by light. This has created a new field that is attracting remarkable attention because of both the scientific interest and its potential applications, such as the coherent control of the precession of a single spin [1] or spin ensemble [2] , [3] , [4] , [5] , [6] , [7] , [8] . Several experiments have revealed a wide variety of physics within this context, for example, ultrafast control through a nonlinear optical process [2] or by employing the magnetic component of terahertz (THz) electromagnetic pulses [9] , [10] . Previous studies focused primarily on the control of the phase and amplitude of a single magnetic oscillation mode. In this case, the three-dimensional trajectory of magnetization motion cannot be altered. As a next step, we propose a new technique to control magnetization in a multidimensional space to fully employ its vectorial properties. This technique can lead to further applications, such as storing multiple pieces of information in a single storage element and the implementation of novel quantum processing using light-spin interactions. 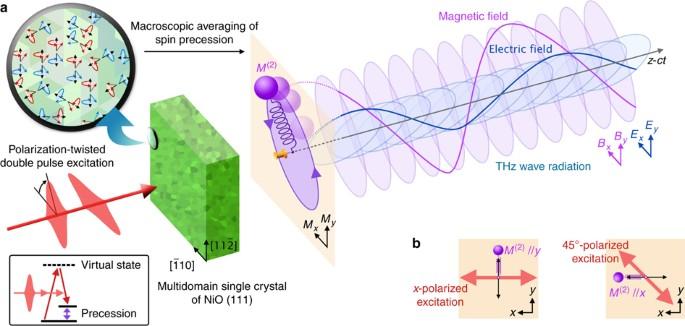Figure 1: Schematic illustrations of the experiment. (a) Vectorial magnetic oscillation control and the resultant THz radiation by double-pulse excitation. The precession motions of the spins are induced in a multidomain single crystal of NiO via a stimulated Raman-type nonlinear optical process, as shown in the inset. Spin motions result in a macroscopic magnetization vector (M(2)) that behaves as an isotropic harmonic oscillator. By changing the interval and polarization of the incident laser pulses, an arbitrary trajectory of the magnetic oscillations is obtained. (b) Two orthogonal magnetic oscillation modes are labelledxandyin this NiO crystal. They are selectively kicked by tuning the polarization azimuth of the excitation light pulse. To realize such vectorial control, it is necessary to independently address the phase and amplitude of multiple degenerate modes that constitute complete bases for describing magnetization vector dynamics, as shown in Figure 1a . For example, consider a magnetization vector that behaves as an isotropic harmonic oscillator in a two-dimensional space. The motion of the magnetization is described by a linear combination of two degenerate orthogonal modes labelled x and y ( Fig. 1b ), and their relative phases and amplitudes determine its trajectory. Figure 1: Schematic illustrations of the experiment. ( a ) Vectorial magnetic oscillation control and the resultant THz radiation by double-pulse excitation. The precession motions of the spins are induced in a multidomain single crystal of NiO via a stimulated Raman-type nonlinear optical process, as shown in the inset. Spin motions result in a macroscopic magnetization vector ( M (2) ) that behaves as an isotropic harmonic oscillator. By changing the interval and polarization of the incident laser pulses, an arbitrary trajectory of the magnetic oscillations is obtained. ( b ) Two orthogonal magnetic oscillation modes are labelled x and y in this NiO crystal. They are selectively kicked by tuning the polarization azimuth of the excitation light pulse. Full size image Here we demonstrate a full manipulation of two-dimensional magnetic oscillations in an antiferromagnetic NiO crystal by employing a pair of polarization-twisted optical pulses. This technique opens new horizons for the optical manipulation of magnetization vectors. Excitation and detection of oscillating magnetization in NiO To demonstrate this vectorial control of magnetization, an as-grown single crystal of antiferromagnetic NiO (111), which has a micro-multidomain structure, is an excellent candidate. Here we employed Raman-type nonlinear optical processes to excite magnetic oscillations [2] , [11] , [12] , [13] and terahertz time-domain spectroscopy (THz–TDS) to detect these oscillations [14] . This combination of material and techniques has several advantages, as described below. First, the magnetic susceptibility of this multidomain sample is defined by a scalar quantity, because macroscopic averaging of the magnetization over domains is valid, as examined by linear absorption measurements [15] . In addition, the absorption spectrum exhibits a sharp peak in the proximity of the antiferromagnetic resonance [16] . Thus, this macroscopic magnetization behaves as an isotropic harmonic oscillator with respect to the linear optical response. Second, because of its strong exchange field and high Néel temperature ( T N =523 K), the resonant frequency Ω mag is as high as ~1 THz at room temperature. This mode is infrared-active [17] , [18] , and this resonant frequency is well within the scope of THz–TDS [14] , [15] , [19] . Therefore, we can directly obtain the magnetization trajectory that is projected on a plane by observing the polarization states of the THz wave that is radiated from the oscillations through a magnetic dipole radiation process [20] . The electric field E ( Ω ) that is radiated from the oscillating magnetization M ( Ω ) at a frequency Ω can be described as: where ɛ , χ μ and k are the permittivity, magnetic linear susceptibility and wave vector of the radiation, respectively. Under irradiation by short laser pulses with broadband spectra, magnetization is induced according to the following equation [21] : where E ( ω ) is the Fourier component of the electric field of the excitation optical pulse at a frequency ω , M (2) ( Ω ) is the Fourier component of the second-order nonlinear magnetization at a frequency Ω and χ ijk (2)MEE is the third-rank, axial time-odd tensor that describes the nonlinear susceptibility. In this Raman process, magnetic oscillations are impulsively excited within the pulse duration of ~100 fs, which is much shorter than an oscillation cycle. Therefore, by changing the laser pulse timing, the phase of an oscillation mode can be changed, as we demonstrated by coherently controlling a magnetic oscillation mode by double-pulse excitation. It is important to note that this nonlinear optical process does not induce excess heating because the light carries away the extra energy that corresponds to the energy mismatch between the magnetic oscillations (~1 meV) and light (~1 eV). They coherently interact with one another, following well-defined polarization selection rules that have been determined by the symmetry of the crystal [22] . As stated above, the effective medium approximation is valid for multidomain NiO. As a result, the system possesses a threefold rotational symmetry around the [111] axis. Although this symmetry assures the isotropic linear optical responses, the nonlinear optical response is not isotropic [23] , and the direction of the excited magnetic oscillations is determined by the polarization angle of the excitation laser pulse [15] . Thus, the two degenerate modes can be independently controlled, as we discuss below in detail. The coherent control of magnetization Figure 1 depicts a schematic representation of the experiment. Ti:sapphire-based femtosecond laser pulses were employed as the pumping beam, which propagated along the [111] axis of an as-grown bulk single crystal of NiO. The pump pulses were separated into a pair of pulses, wherein the pulse interval and polarization angles were controlled. The polarization properties of the THz electromagnetic waves that radiated from the induced dynamic magnetization were studied via the electro-optic sampling method [14] and the THz polarimetry technique using a pair of wire-grid polarizers [24] (Methods). All measurements were performed at room temperature. Employing double-pulse excitation, we performed the coherent control [25] , [26] of a magnetic oscillation mode, as shown in Figure 1a , in which the polarization angles of the two pulses are the same ( Fig. 2a ). The decay time of this magnetic resonance was on the order of tens of picoseconds [15] , [19] , which was much longer than a cycle of the magnetic oscillations. Within this coherence time, we could superpose the magnetic oscillations that were induced by the first and second pulses. The amplitude of the THz signal after the excitation by the second pulse periodically changed as a function of the time interval τ between the pulses ( Fig. 2b ). Each of the two optical pulses induces monochromatic magnetic oscillations with the antiferromagnetic resonance frequency. Therefore, Ω mag τ determines the phase difference between these oscillations that have been created by the two optical pulses. When Ω mag τ / π was an even integer, they constructively interfered, resulting in an enhancement of the amplitude of the THz signal ( Fig. 2c ). In contrast, when Ω mag τ / π was an odd integer, they destructively interfered, and the magnetization was cancelled ( Fig. 2d ). 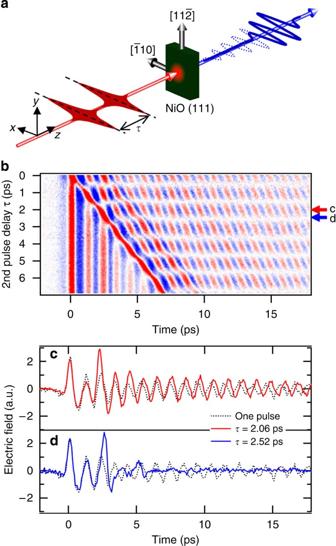Figure 2: Coherent control of the magnetization oscillations in NiO using linearly polarized double-pulse excitation with the same polarization angle. (a) Schematic illustrations of the experiment concerning coherent control with double-pulse excitation, wherein both pulses are linearly polarized along thex-axis. The intervalτbetween the two pulses can be tuned. (b) Two-dimensional plot of the time-domain THz signal. The signs (+/0/−) and amplitudes of the electric fields are expressed by colours (red/white/blue) and their shades. The periodically aligned horizontal white lines correspond to the suppression of the spin motion by the destructive interference between two two-excitation pulse-induced waves. Temporal profiles at fixed values ofτare shown in c and d. The two waves constructively (c) or destructively (d) interfere with one another. Figure 2: Coherent control of the magnetization oscillations in NiO using linearly polarized double-pulse excitation with the same polarization angle. ( a ) Schematic illustrations of the experiment concerning coherent control with double-pulse excitation, wherein both pulses are linearly polarized along the x -axis. The interval τ between the two pulses can be tuned. ( b ) Two-dimensional plot of the time-domain THz signal. The signs (+/0/−) and amplitudes of the electric fields are expressed by colours (red/white/blue) and their shades. The periodically aligned horizontal white lines correspond to the suppression of the spin motion by the destructive interference between two two-excitation pulse-induced waves. Temporal profiles at fixed values of τ are shown in c and d. The two waves constructively ( c ) or destructively ( d ) interfere with one another. Full size image The vectorial control of magnetization We extended this technique to the arbitrary control of the trajectory of the magnetic oscillations, that is, the independent control of the two degenerate modes. Before discussing this experiment, note that such arbitrary control cannot be realized by a single excitation pulse with a fixed polarization, although a plane wave of light has the same number of parameters as the two-dimensional motion of magnetization. This is because the information of the carrier phase of the light was lost in the Raman process, decreasing the number of control parameters. In the case of multidomain NiO (111), the non-vanishing transverse components of the nonlinear susceptibility tensor χ ijk (2)MEE ( Ω ;− ω , ω+Ω ) are χ yxx (2)MEE =− χ yyy (2)MEE = χ xxy (2)MEE = χ xyx (2)MEE ≡ α ( Ω , ω ). Equation (2) is reduced to the following: When the incident laser has a fixed polarization, that is, the ratio between the complex amplitudes of the electric fields E x ( ω ): E y ( ω ) does not depend on ω , M x and M y are always real-valued quantities, according to this equation. Thus, the relative phase of the two orthogonal oscillations cannot be tuned. The result is that the THz wave that is radiated from M (2) is always linearly polarized. On the other hand, the direction of the oscillation can be tuned by changing the polarization azimuthal angle φ of the incident laser with respect to the x -axis ([−110] axis of the crystal), where E x ( ω )= E ( ω ) cos φ , E y ( ω )= E ( ω ) sin φ , and equation (3) is reduced to To handle the relative phase of the two basis modes, we employed a pair of linearly polarized laser pulses with different polarization angles. As determined from equation (4), the azimuthal angle of the induced magnetic oscillation changed by −2Δ φ when φ changed by Δ φ . This polarization angle dependence was generally valid when the system had a threefold rotational symmetry. Therefore, two orthogonal oscillation modes can be independently accessed, if the angle between the azimuths of the two pulses is 45° ( Fig. 3a ). By changing the interval between these two pulses, the relative phase of the oscillation modes is controlled because the oscillation is instantaneously kicked within the ultrashort duration of a laser pulse. 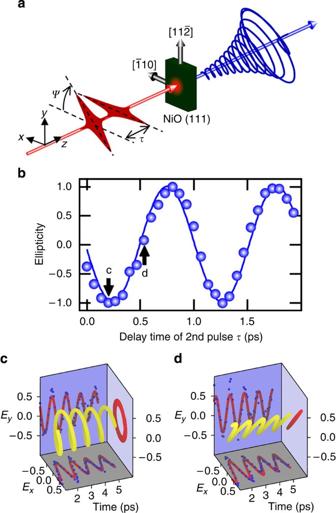Figure 3: Vectorial magnetization control with polarization-twisted double-pulse excitation. (a) Schematic illustrations of the vectorial control of the magnetization vector. Both pulses are linearly polarized. The first is polarized along thex-axis, whereas the second has an azimuthal angle ofψψ. By properly tuningτandψψ, we can manipulate the motion of the magnetization vector to follow an arbitrarily designed direction and amplitude of polarization. (b) Ellipticity of the measured THz radiation atΩmagas a function of the intervalτbetween the two linearly polarized excitation pulses. The first pulse isx-polarized, whereas the polarization azimuth of the second is 45° with respect to thex-axis. Any ellipticity between the purely right and left circular polarizations is obtained by tuningτ. The solid curve is a fit of the data by a sine curve. The three-dimensional trajectories of the electric field vectors with fixed values ofτare shown in (c,d). The radiation is purely circularly polarized (c) or linearly polarized (d). The dots correspond to the projections of the experimental data onto thex- andy-axes. The solid curves correspond to the fit of exponentially decaying sine functions; the phase differences between thex- andy-components are determined byΩmagτ/π. Figure 3b shows the measured ellipticity (| M r | − | M l |)/(| M r | + | M l |) as a function of the delay time τ , where M r and M l are the right and left circular components of M , respectively. The polarization of the THz wave that was radiated from M was circular when it was a half-integer ( Fig. 3c ) and was linear when Ω mag τ / π was an integer ( Fig. 3d ). We continuously changed the ellipticity from −1 to +1 by sweeping τ . Note that the selective excitation of circularly polarized magnetization is possibly independent of the crystal azimuthal orientation. Figure 3: Vectorial magnetization control with polarization-twisted double-pulse excitation. ( a ) Schematic illustrations of the vectorial control of the magnetization vector. Both pulses are linearly polarized. The first is polarized along the x -axis, whereas the second has an azimuthal angle of ψψ . By properly tuning τ and ψψ , we can manipulate the motion of the magnetization vector to follow an arbitrarily designed direction and amplitude of polarization. ( b ) Ellipticity of the measured THz radiation at Ω mag as a function of the interval τ between the two linearly polarized excitation pulses. The first pulse is x -polarized, whereas the polarization azimuth of the second is 45° with respect to the x -axis. Any ellipticity between the purely right and left circular polarizations is obtained by tuning τ . The solid curve is a fit of the data by a sine curve. The three-dimensional trajectories of the electric field vectors with fixed values of τ are shown in ( c , d ). The radiation is purely circularly polarized ( c ) or linearly polarized ( d ). The dots correspond to the projections of the experimental data onto the x - and y -axes. The solid curves correspond to the fit of exponentially decaying sine functions; the phase differences between the x - and y -components are determined by Ω mag τ / π . Full size image We demonstrate a method for the all-optical manipulation of the dynamics of a magnetization vector in NiO. By designing timing- and polarization-tuned, double-pulse excitation, selective manipulation of two degenerate oscillation basis modes was achieved on the basis of well-defined polarization selection rules. In particular, a simple change of the interval between two laser pulses selectively induced clockwise or anticlockwise rotational motion of the magnetization vector. The scope of our technique is not limited to this specific example because the selective control of rotation means that the angular momentum that is transferred from the light to the material is tuned. For example, the initialization of a single spin and selective manipulation of degenerate elementary excitations are promising possible applications. Here the temporal variation of the polarization angle of the incident light has a key role in this technique. Thus, an approach that employs polarization-shaped laser pulses [27] should be further examined. In addition to spintronics applications, this technique has potential in THz technology, wherein the control of elementary excitations that fall in the THz spectral range is of particular interest. Materials An as-grown single crystal of NiO (111) with a thickness of 100 μm was used for this study. The direction of the spin ordering and associated lattice distortions resulted in 12 types of domains in this crystal, which were randomly distributed in the as-grown sample with the same population, as described below. NiO crystallizes in a rocksalt structure, and, below its Néel temperature T N =523 K, the spins are ordered ferromagnetically in the {111} plane such that the alternate stacking of these layers forms an antiferromagnetic structure [28] . Because of this magnetic ordering, slight rhombohedral distortions were induced along the diagonals; [111] and three other equivalents, which were accommodated by twin structures, formed four kinds of T-domains. Experimentally, the T-domains were distinguished by the birefringence because of their lattice distortions. The sizes of the T-domains in our sample were smaller than 10 μm, according to polarization microscopy. In each T-domain, three equivalent spin orientations formed three types of S-domains; thus, there were 12 types of domains in total. For example, in the T 1 -domain, in which spins were ordered in the (111) plane, the spins were aligned along the [11–2], [1–21] or [−211] directions. These S-domains were also randomly distributed, and they were typically smaller than 1 μm [29] . In this micro-multidomain sample, a sharp antiferromagnetic resonance in the vicinity of ~1 THz was identified by absorption measurements that employed THz–TDS. No other resonance was observed in the spectral range of 0.5–2 THz. The linear absorption exhibited no dependence on the polarization of the incident THz wave, that is , there was neither birefringence nor chirality in the THz range. In our experimental conditions, the effects of phase mismatch were negligible because the coherent length of the nonlinear optical interaction was 130 μm, which exceeded the sample thickness (100 μm), and because the refractive indices of NiO for the THz wave and fundamental excitation light were 3.5 and 2.3, respectively [30] . Note that the absorption coefficient of NiO at 800 nm was small [31] , and we could thus eliminate indirect magnon generation processes through one-photon absorption followed by thermal relaxation processes. Experimental setup A Ti:sapphire-based regenerative amplifier was used as a light source. The central wavelength was 800 nm, the pulse duration was 140 fs and the repetition rate was 1 kHz. The beam was divided into two beams and used as a pump beam for the sample excitation and as a probe beam for the electro-optic sampling. The spot size of the excitation onto the sample was approximately 1 mm in diameter, which is much larger than the single domain size (~10 μm); hence, the coherent superposition of the signals that were generated in each of the domains was valid. The pulse energy was less than ~300 μJ. The THz wave radiation was collected with parabolic mirrors, and the electric field was detected via the electro-optic sampling method using a 1-mm-thick ZnTe (110) crystal. The electric field vector of the THz radiation was obtained via THz polarimetry using two wire-grid polarizers [24] . How to cite this article: Kanda, N. et al . The vectorial control of magnetization by light. Nat. Commun. 2:362 doi: 10.1038/ncomms1366 (2011).